Large-scale reorganization of the somatosensory cortex following spinal cord injuries is due to brainstem plasticity Adult mammalian brains undergo reorganization following deafferentations due to peripheral nerve, cortical or spinal cord injuries. The largest extent of cortical reorganization is seen in area 3b of the somatosensory cortex of monkeys with chronic transection of the dorsal roots or dorsal columns of the spinal cord. These injuries cause expansion of intact face inputs into the deafferented hand cortex, resulting in a change of representational boundaries by more than 7 mm. Here we show that large-scale reorganization in area 3b following spinal cord injuries is due to changes at the level of the brainstem nuclei and not due to cortical mechanisms. Selective inactivation of the reorganized cuneate nucleus of the brainstem eliminates observed face expansion in area 3b. Thus, the substrate for the observed expanded face representation in area 3b lies in the cuneate nucleus. Massive deafferentation due to spinal cord injuries in adult primates results in large-scale changes in the brain organization. For example, following lesions of the dorsal columns of the spinal cord, face inputs expand into the deafferented hand representation of the primary somatosensory area 3b, shifting the representational boundaries by 7–14 mm (refs 1 , 2 , 3 , 4 ) and sometimes more [2] . Such large-scale expansion of chin inputs into the deafferented hand region was first described in adult macaque monkeys [5] that had undergone transection of the dorsal roots from C2 to T4. This kind of reorganization is seen in many other parts of the brain including second somatosensory and parietal ventral areas of the somatosensory cortex [3] and the ventroposterior lateral nucleus (VPL) of the thalamus [2] , [4] . Brain reorganization causes perceptual abnormalities such as phantom sensations and phantom pain [6] , [7] , [8] , [9] and also has implications for recoveries from such injuries [10] . However, mechanisms of brain reorganization are not known. Interconnections between the hand and the face representations along the dorsal column-medial lemniscal pathway are absent or extremely restricted [11] , [12] , [13] , [14] . Therefore, the reorganization is unlikely to be due to unmasking or potentiation of previously existing but silent connections that can occur when the primary afferent drive is removed [15] , [16] . The plastic changes are, therefore, likely to be mediated by axonal sprouting [13] , or withdrawal of synapses and neuronal degeneration following deafferentations [17] . The mechanisms that lead to brain reorganization can operate at the cortical [18] , [19] , thalamic [17] , [20] or brainstem levels [4] , [21] , [22] , or even at multiple sites [13] ( Fig. 1 ). In the cortex there is evidence that axonal sprouting plays a role in visuotopic reorganization following retinal lesions [23] , [24] . Sprouting also accompanies expansion of stump representation in the somatosensory cortex following limb amputations [25] and plasticity of the motor cortex [26] . In the brainstem nuclei sprouting of inputs from the trigeminal nucleus into the cuneate nucleus has been shown following dorsal column injuries [22] . Degenerative changes in the cortex, thalamus and cuneate nucleus are observed in monkeys with long-term loss of sensory inputs [20] , [27] . Thus, mechanisms operating at any one or all of these sites along the somatosensory pathway could potentially contribute to cortical reorganization. However, no causal relationship between any of these changes and cortical reorganization has been shown. 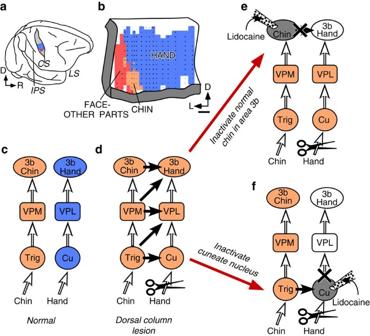Figure 1: Possible mechanisms of large-scale brain reorganization and the experimental design. (a) Location of area 3b in the posterior bank of the central sulcus is shown on an outline diagram of the macaque brain. Central sulcus (CS) is drawn partially opened. D, dorsal; IPS, intraparietal sulcus; LS, lateral sulcus; R, rostral. (b) Normal somatotopy in area 3b showing representation of the hand (blue), chin (orange) and other parts of the face (red) onen faceview of the posterior bank of CS reconstructed from histological sections of the brain. Dots mark locations of the recording sites where receptive fields of the neurons were mapped (see ‘Methods’). Scale bar, 1 mm. (c) In normal monkeys inputs from the chin ascend to area 3b via the trigeminal nucleus of the brainstem (Trig) and the ventroposterior medial nucleus (VPM) of the thalamus. Inputs from the hand ascend via cuneate nucleus (Cu) and the ventroposterior lateral nucleus (VPL). (d) In monkeys with chronic lesions of the dorsal columns, neurons in the deafferented hand region of area 3b1, VPL2and cuneate nucleus (this study) respond to touch on the chin. Possible mechanisms include growth between the normal chin inputs and the deafferented hand regions at the cortical, thalamic or brainstem levels (black arrows)13. (e) Inactivation of the normal chin region in area 3b would silence the expanded chin representation if cortical growth is the primary cause for area 3b reorganization. (f) If area 3b reorganization is due to upstream effects of growth at the medullary level, inactivation of the reorganized cuneate nucleus would render silent the expanded chin representation in area 3b. Figure 1: Possible mechanisms of large-scale brain reorganization and the experimental design. ( a ) Location of area 3b in the posterior bank of the central sulcus is shown on an outline diagram of the macaque brain. Central sulcus (CS) is drawn partially opened. D, dorsal; IPS, intraparietal sulcus; LS, lateral sulcus; R, rostral. ( b ) Normal somatotopy in area 3b showing representation of the hand (blue), chin (orange) and other parts of the face (red) on en face view of the posterior bank of CS reconstructed from histological sections of the brain. Dots mark locations of the recording sites where receptive fields of the neurons were mapped (see ‘Methods’). Scale bar, 1 mm. ( c ) In normal monkeys inputs from the chin ascend to area 3b via the trigeminal nucleus of the brainstem (Trig) and the ventroposterior medial nucleus (VPM) of the thalamus. Inputs from the hand ascend via cuneate nucleus (Cu) and the ventroposterior lateral nucleus (VPL). ( d ) In monkeys with chronic lesions of the dorsal columns, neurons in the deafferented hand region of area 3b [1] , VPL [2] and cuneate nucleus (this study) respond to touch on the chin. Possible mechanisms include growth between the normal chin inputs and the deafferented hand regions at the cortical, thalamic or brainstem levels (black arrows) [13] . ( e ) Inactivation of the normal chin region in area 3b would silence the expanded chin representation if cortical growth is the primary cause for area 3b reorganization. ( f ) If area 3b reorganization is due to upstream effects of growth at the medullary level, inactivation of the reorganized cuneate nucleus would render silent the expanded chin representation in area 3b. Full size image Here we determined the extent to which mechanisms operating at different levels potentially contribute to the cortical plasticity in macaque monkeys with unilateral lesions of the dorsal columns at cervical levels. We first show that corticocortical mechanisms do not contribute to cortical plasticity. We then show that reorganization of the cuneate nucleus of the brainstem is the critical change that is required for manifestation of large-scale brain plasticity. Expansion of the chin representation in area 3b, and perhaps in the VPL of thalamus and the rest of the brain, is an upstream reflection of the reorganization of the brainstem nuclei. Large-scale plasticity is not due to cortical mechanisms We first determined whether in monkeys with dorsal column lesions expansion of chin representation into the deafferented hand region of area 3b is mediated by cortical mechanisms. We hypothesized that, if expansion of the chin inputs into the deafferented hand region of area 3b is due to growth from the normal chin representation, inactivation of the normal chin region would silence the medially expanded chin representation ( Fig. 1 ). We tested this hypothesis in three macaque monkeys LM76 ( Macaca mulatta ), LM95 ( Macaca radiata ) and LM105 ( Macaca mulatta ) with chronic unilateral lesions of the dorsal columns. In monkey LM76, we mapped the contralesional area 3b (see Methods and ref. 3 ) 20 months after transection of the left dorsal columns at C5 level ( Fig. 2 ). The data revealed that the chin responsive region had expanded into the deafferented hand cortex as far medial as the cortex was mapped, a distance of 7 mm ( Fig. 2a ; compare with Fig. 1b ). Responses to stimulation of the chin were evoked at 95.7% ( n =111) of the responsive sites medial to the hand-face border. At all the recording sites in the expanded chin representation, receptive fields were on the rostral part of the chin ( Fig. 2c ; Fig. 3 ). At few sites, neurons also responded to stimulation of the skin on the hand or the arm, likely due to minor sparing of the dorsal column fibres and the segmental level of the lesion [2] . 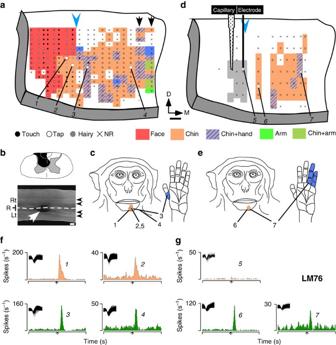Figure 2: Inactivating normal chin representation in area 3b does not affect chin expansion. (a) Somatotopy in area 3b of monkey LM76 with chronic dorsal column lesion. Neurons in the deafferented hand region respond to touch on the chin, shown in orange. Light blue arrowhead marks location of the hand-face border. At some of the sites, neurons responded to touch on both the hand and the chin because the lesion was partial (see the colour code). Black arrows on top mark the electrode penetrations illustrated in Fig. 3. Scale bar, 1 mm. (b) Top, reconstruction of the spinal cord in a coronal plane to show extent of the spinal cord lesion. Bottom, dark-field photomicrograph of a horizontal section of the spinal cord showing the lesion site (white arrow). The white dashed line marks the midline; black arrows mark boundaries of the grey matter. Lt, Left; R, rostral; Rt, right; Scale bar, 1 mm. (c) Location of chin receptive fields at sites marked as 1 to 4 in ‘a’ and 5 in ‘c’. (d) Site of the lidocaine injection in the normal chin representation using a capillary tube attached to an electrode. Region of the normal chin representation, shown in grey, is transposed from ‘a’ for reference. After lidocaine infusion, neuronal responses in the normal chin representation were not evoked, whereas responses to chin stimulation in the deafferented hand region were not affected. (e) Location of the post-inactivation chin receptive fields at sites marked as 6 and 7 in ‘d’. Receptive field for the site 5 was same as ‘2’ shown in ‘c’, because they are the same recording site. (f) Peristimulus time histograms (PSTH) showing multiunit responses to tactile stimulation of the chin (see ‘Methods’). Graphs show neuronal responses recorded at the corresponding sites marked in ‘a’. Recording sites 1 and 2 were in the normal chin region, and 3 and 4 in the expanded chin representation. Thex-axis range is from 100 ms before the stimulation onset (arrow) to 100 ms post-stimulus onset. Insets show the waveforms. (g) PSTH showing multiunit responses after lidocaine infusion at sites 5, 6 and 7 shown in ‘d’. Figure 2: Inactivating normal chin representation in area 3b does not affect chin expansion. ( a ) Somatotopy in area 3b of monkey LM76 with chronic dorsal column lesion. Neurons in the deafferented hand region respond to touch on the chin, shown in orange. Light blue arrowhead marks location of the hand-face border. At some of the sites, neurons responded to touch on both the hand and the chin because the lesion was partial (see the colour code). Black arrows on top mark the electrode penetrations illustrated in Fig. 3. Scale bar, 1 mm. ( b ) Top, reconstruction of the spinal cord in a coronal plane to show extent of the spinal cord lesion. Bottom, dark-field photomicrograph of a horizontal section of the spinal cord showing the lesion site (white arrow). The white dashed line marks the midline; black arrows mark boundaries of the grey matter. Lt, Left; R, rostral; Rt, right; Scale bar, 1 mm. ( c ) Location of chin receptive fields at sites marked as 1 to 4 in ‘ a ’ and 5 in ‘ c ’. ( d ) Site of the lidocaine injection in the normal chin representation using a capillary tube attached to an electrode. Region of the normal chin representation, shown in grey, is transposed from ‘ a ’ for reference. After lidocaine infusion, neuronal responses in the normal chin representation were not evoked, whereas responses to chin stimulation in the deafferented hand region were not affected. ( e ) Location of the post-inactivation chin receptive fields at sites marked as 6 and 7 in ‘ d ’. Receptive field for the site 5 was same as ‘2’ shown in ‘ c ’, because they are the same recording site. ( f ) Peristimulus time histograms (PSTH) showing multiunit responses to tactile stimulation of the chin (see ‘Methods’). Graphs show neuronal responses recorded at the corresponding sites marked in ‘ a ’. Recording sites 1 and 2 were in the normal chin region, and 3 and 4 in the expanded chin representation. The x -axis range is from 100 ms before the stimulation onset (arrow) to 100 ms post-stimulus onset. Insets show the waveforms. ( g ) PSTH showing multiunit responses after lidocaine infusion at sites 5, 6 and 7 shown in ‘ d ’. 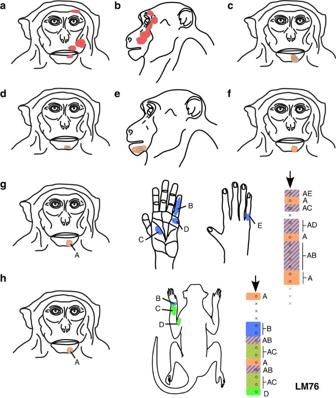Figure 3: Examples of receptive fields of neurons in area 3b of monkey LM76. (a,b) Receptive fields of neurons in the normal face region, other than the chin. (c–e) Examples of receptive fields in the normal chin representation. (f) The chin region encompassed by all the receptive fields of neurons in the expanded chin representation. The receptive fields were restricted to the rostral part of the chin (seeFig. 2). (g,h) Examples of receptive fields of neurons encountered in two penetrations marked by black arrowheads inFig. 2a. Neurons at some of the recording sites had dual receptive fields on the hand and the chin due to sparing of the dorsal column fibres. Full size image Figure 3: Examples of receptive fields of neurons in area 3b of monkey LM76. ( a , b ) Receptive fields of neurons in the normal face region, other than the chin. ( c – e ) Examples of receptive fields in the normal chin representation. ( f ) The chin region encompassed by all the receptive fields of neurons in the expanded chin representation. The receptive fields were restricted to the rostral part of the chin (see Fig. 2 ). ( g , h ) Examples of receptive fields of neurons encountered in two penetrations marked by black arrowheads in Fig. 2a . Neurons at some of the recording sites had dual receptive fields on the hand and the chin due to sparing of the dorsal column fibres. Full size image We then infused lidocaine (4%), a sodium channel blocker, in the normal chin representation of area 3b, ~1.25 mm lateral to the hand-face border, using a fine capillary tube attached to a syringe pump (see Methods). An independently moveable electrode was attached to the capillary tube to continuously monitor neuronal responses in the vicinity of the electrode throughout the experiment. Evoked neuronal responses in the normal chin region were abolished 12 min after start of the lidocaine infusion. However, even though the normal chin inputs to area 3b were inactivated, somatotopic mapping revealed that neurons in the deafferented hand cortex continued to respond to tactile stimulation of the chin ( Fig. 2d ). Neuronal responses to chin stimulation were observed at 100% ( n =29) of the sites that were mapped medial to the expected hand-face border. Similar results were obtained from the other two monkeys, LM95 and LM105, mapped 2 and 3 years after lesion of the dorsal columns. In all the three monkeys, neuronal responses were quantified by recording multiunit activity using tungsten microelectrodes. The receptive fields on the chin were stimulated using a Chubbuck type electromechanical vibratory stimulator (at 1 Hz; skin contact time 10 ms per cycle; see Methods). The data showed that lidocaine infusion in the normal chin region did not affect neuronal responses to chin stimulation in the expanded chin representation (in the three monkeys mean peak firing rate before inactivation was 75.8 spikes s −1 , n =18; after inactivation 63.6 spikes s −1 , n =11; P =0.406, Mann–Whitney rank sum test; Fig. 2f,g ). Simultaneous recordings from the normal chin region confirmed absence of any detectable evoked responses in the normal chin region ( Fig. 2f,g ). Results from these experiments show that normal chin inputs to area 3b are not essential for expression of emergent chin responses in the deafferented hand region of area 3b. This suggests that sprouting of normal chin inputs of area 3b into the deafferented parts of the cortex does not mediate large-scale brain reorganization. The likely sites of the origin of plasticity would therefore be the VP nucleus of the thalamus and/or the brainstem nuclei ( Fig. 1d ) [13] , [17] , [21] . Cortical plasticity reflects reorganized cuneate inputs We determined whether expansion and expression of chin inputs into the cuneate nucleus is essential for the reorganization observed in area 3b. Two macaque monkeys LM49 ( Macaca radiata ) and LM59 ( Macaca mulatta ) were used for these experiments. In monkey LM49, 14 months after transection of the left dorsal columns at C4/C5 level, we mapped contralesional area 3b to determine the extent of chin expansion. As expected, neuronal responses to the chin stimulation were observed in the entire mapped extent of the deafferented hand cortex (7.1 mm; Fig. 4a ). Responses to stimulation of the chin were evoked at 100% ( n =159) of the responsive sites in the deafferented hand cortex. 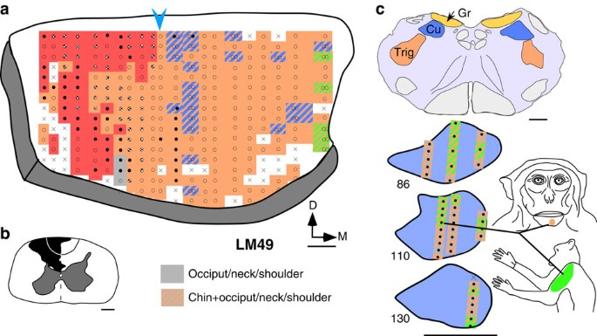Figure 4: Somatotopy in the cuneate nucleus and area 3b in monkey LM49 with chronic lesion of the dorsal columns. (a) Reorganized somatotopy in area 3b showing expansion of the chin responsive area. (b) Reconstruction of the spinal cord lesion site showing extent of the lesion. (c) An outline diagram of a coronal section of the medulla showing locations of the cuneate (Cu), spinal trigeminal (Trig) and gracile (Gr) nuclei. Shown below is the somatotopy along seven electrode tracks through three rostrocaudal levels of the cuneate nucleus of monkey LM49 with chronic lesion of the dorsal columns. Receptive fields at most of the recording sites were either on the chin (orange) or on the arm (green) and shoulder. Dual receptive field at one of the sites is illustrated. The numbers below refer to the section numbers, each section was 36 μm thick. D, dorsal; M, medial. Scale bars, 1 mm. For other conventions seeFig. 2. Figure 4: Somatotopy in the cuneate nucleus and area 3b in monkey LM49 with chronic lesion of the dorsal columns. ( a ) Reorganized somatotopy in area 3b showing expansion of the chin responsive area. ( b ) Reconstruction of the spinal cord lesion site showing extent of the lesion. ( c ) An outline diagram of a coronal section of the medulla showing locations of the cuneate (Cu), spinal trigeminal (Trig) and gracile (Gr) nuclei. Shown below is the somatotopy along seven electrode tracks through three rostrocaudal levels of the cuneate nucleus of monkey LM49 with chronic lesion of the dorsal columns. Receptive fields at most of the recording sites were either on the chin (orange) or on the arm (green) and shoulder. Dual receptive field at one of the sites is illustrated. The numbers below refer to the section numbers, each section was 36 μm thick. D, dorsal; M, medial. Scale bars, 1 mm. For other conventions see Fig. 2 . Full size image We then mapped the brainstem nuclei of this monkey to determine whether the cuneate nucleus, which normally receives inputs from the hand and the arm, also undergoes large-scale reorganization. Expansion of face representation into the cuneate nucleus of monkeys with chronic deafferentation has not been described before. We made 11 electrode penetrations through the rostrocaudal extent of the cuneate nucleus. Neurons responded to touch on the chin at 85.5% of the recording sites ( n =62), although at most of these site responses to stimulation of the arm or shoulder were also present ( Fig. 4c ). Of the remaining sites, neurons at one site had receptive field on the arm, at one site on the shoulder, and at seven sites no responses were observed to touch on any part of the body. All the emergent face receptive fields in the cuneate nucleus were on the rostral chin ( Fig. 4c ), a skin region innervated by mandibular branch of the trigeminal nerve [28] . The chin receptive fields in the cuneate nucleus were similar to the chin receptive fields in the reorganized area 3b. Neurons in the cuneate nucleus normally do not respond to tactile stimulation of the chin [29] , [30] , [31] . In next part of the experiment we placed an array of eight tungsten microelectrodes in area 3b to simultaneously record from the normal chin and the expanded chin representations ( Fig. 5 ). Two of the electrodes, separated by 350 μm, were in the normal chin region, and six electrodes, covering 3.3 mm of the cortex, were in the deafferented hand region ( Fig. 5a ). Simultaneous neuronal recordings were done from the cuneate nucleus ( Fig. 5d ) and area 3b ( Fig. 5g ) while stimulating receptive fields on the chin ( Fig. 5c ; 1 Hz; skin contact time 10 ms per cycle; see Methods). We then inactivated neurons in the cuneate nucleus by injecting lidocaine using a fine capillary tube (see Methods). Lidocaine was injected at four sites spanning 3 mm rostrocaudally, at a depth of 700–1,500 μm from the surface of the medulla (2 or 4 μl per site at 4 μl min −1 ). Total time for completing all the four injections was 13 min. The capillary was removed and recording electrodes were placed in the cuneate and the spinal trigeminal nuclei to ascertain that neurons in the cuneate nucleus were inactivated ( Fig. 5e ) whereas the adjacent trigeminal nucleus was not affected ( Fig. 5f ). Recordings from the electrode array in area 3b revealed that inactivation of the cuneate nucleus completely abolished neuronal responses to chin stimulation in the deafferented hand region of area 3b ( Fig. 5h ) without affecting responses in the normal chin representation (mean peak firing rate before inactivation, 159.8 spikes s −1 ; mean peak firing rate post-inactivation, 165.7 spikes s −1 ; P =1.0, Mann–Whitney rank sum test, n =3). Throughout the recording session, activity in the cuneate nucleus was simultaneously monitored to ensure that it remained inactivated. 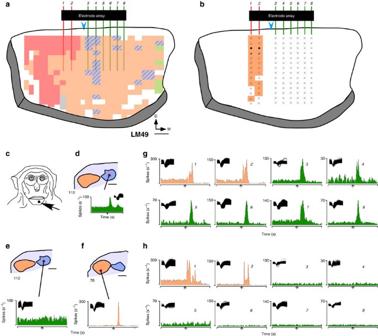Figure 5: Inactivation of the cuneate nucleus abolished observed cortical reorganization in monkey LM49. (a) Approximate locations of the electrode tips of the 8-electrode array (see ‘Methods’). For reference somatotopic map transposed fromFig. 4ais shown in low key. (b) Reconstruction of the posterior bank of the central sulcus showing that neuronal responses in the normal chin representation were not affected by lidocaine infusion in the cuneate nucleus. However, responses to tactile stimulation of the chin were not evoked in the deafferented hand area at any of the mapped sites. Recordings were done by moving the electrode array through the depth of the sulcus. (c) Location of the stimulation site on the chin (black dot) during recordings for graphs shown in panels ‘d–h’ (d) PSTH and waveforms of multiunit responses to stimulation of the chin at a recording site in the cuneate nucleus (blue) before lidocaine infusion. (e) After inactivation of the cuneate nucleus by lidocaine, neuronal responses to chin stimulation in the cuneate nucleus were abolished. These recordings and those shown in ‘h’ were done simultaneously. (f) Neuronal responses in the adjacent spinal trigeminal nucleus were not affected by injection of lidocaine in the cuneate nucleus. (g) PSTH showing multiunit responses in area 3b to chin stimulation at recording sites shown in ‘a’ before infusion of lidocaine in the cuneate nucleus. (h) Neuronal responses at the same sites after lidocaine infusion. Responses in the normal chin region were intact, while those in the deafferented hand cortex were abolished. They-axis scales for the corresponding graphs in ‘g’ and ‘h’ are same. These recordings and those shown in ‘e’ were done simultaneously. Scale bars, 1 mm. For other conventions seeFig. 2. Figure 5: Inactivation of the cuneate nucleus abolished observed cortical reorganization in monkey LM49. ( a ) Approximate locations of the electrode tips of the 8-electrode array (see ‘Methods’). For reference somatotopic map transposed from Fig. 4a is shown in low key. ( b ) Reconstruction of the posterior bank of the central sulcus showing that neuronal responses in the normal chin representation were not affected by lidocaine infusion in the cuneate nucleus. However, responses to tactile stimulation of the chin were not evoked in the deafferented hand area at any of the mapped sites. Recordings were done by moving the electrode array through the depth of the sulcus. ( c ) Location of the stimulation site on the chin (black dot) during recordings for graphs shown in panels ‘ d – h ’ ( d ) PSTH and waveforms of multiunit responses to stimulation of the chin at a recording site in the cuneate nucleus (blue) before lidocaine infusion. ( e ) After inactivation of the cuneate nucleus by lidocaine, neuronal responses to chin stimulation in the cuneate nucleus were abolished. These recordings and those shown in ‘ h ’ were done simultaneously. ( f ) Neuronal responses in the adjacent spinal trigeminal nucleus were not affected by injection of lidocaine in the cuneate nucleus. ( g ) PSTH showing multiunit responses in area 3b to chin stimulation at recording sites shown in ‘ a ’ before infusion of lidocaine in the cuneate nucleus. ( h ) Neuronal responses at the same sites after lidocaine infusion. Responses in the normal chin region were intact, while those in the deafferented hand cortex were abolished. The y -axis scales for the corresponding graphs in ‘ g ’ and ‘ h ’ are same. These recordings and those shown in ‘ e ’ were done simultaneously. Scale bars, 1 mm. For other conventions see Fig. 2 . Full size image After the neuronal recordings described above were done, area 3b was mapped more extensively. No responses to stimulation of the chin were evoked anywhere in the mapped deafferented hand region ( Fig. 5b ). We continued to monitor neuronal activity in the cuneate nucleus and area 3b until inhibitory effects of lidocaine wore off and responses to tactile stimulation of the chin in the cuneate nucleus returned. We observed that evoked responses to chin stimulation in the deafferented hand region of area 3b also returned simultaneously. In a second monkey, LM59, with lesion of the dorsal columns at C5 level, chin expansion was observed in the cuneate nucleus and area 3b ( Fig. 6 ). Since the lesion of the dorsal columns was nearly complete ( Fig. 6c ), neurons in area 3b responded to touch on the hand at only one recording site ( Fig. 6b ). Multiunit mapping of the cuneate nucleus revealed that neurons responded to chin stimulation at 48% of the recording sites ( n =150, recorded in 22 penetrations through the cuneate nucleus; Fig. 6a ). Out of these, at 12.5% of the sites, we encountered dual receptive fields on the chin and arm, or chin and shoulder/occiput. At the remaining 52% recording sites, neurons either responded to touch on the arm, occiput/shoulder/neck and face, or they were unresponsive. 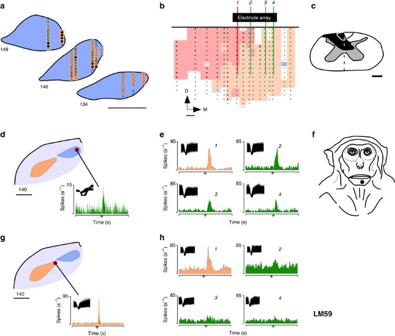Figure 6: Inactivation of the cuneate nucleus abolished responses to chin stimulation in the deafferented parts of area 3b in monkey LM59. (a) Outline drawings of the cuneate nucleus from three different rostrocaudal coronal sections of the medulla showing locations of the receptive fields in 10 different electrode penetrations. Note extensive responses to stimulation on the chin. (b) Approximate locations of the electrode tips in area 3b (see ‘Methods’). For reference somatotopic map derived separately is placed in the background, which also shows expansion of the chin responsive region in the deafferented hand cortex. (c) A reconstruction of the spinal cord in a coronal plane showing the extent of the dorsal column lesion. (d) PSTH and waveforms of neuronal responses to stimulation of the chin at a recording site marked by deep red dot in the cuneate nucleus (blue) before lidocaine infusion. Two responsive units are clearly discernable. (e) PSTH showing multiunit responses in area 3b to chin stimulation at recording sites shown in ‘b’ before infusion of lidocaine in the cuneate nucleus. (f) Location of the stimulation site on the chin (black dot) during recordings for graphs shown in panels ‘d’, ‘e’, ‘g’ and ‘h’. (g) PSTH showing that neuronal responses in the spinal trigeminal nucleus were not affected by injection of lidocaine in the adjacent cuneate nucleus. (h) Neuronal responses at the same sites as for recordings shown in ‘e’ after lidocaine infusion. Responses in the normal chin region were intact, while those in the deafferented hand cortex were abolished. Thex-axis range is from 100 ms before the stimulation onset (arrow) to 100 ms post-stimulus onset for ‘e’ and ‘h’, and from 400 ms pre-stimulus onset to 400 ms post-stimulus onset for ‘d’ and ‘g’. Scale bars, 1 mm. For other conventions seeFigs 2,4and5. Figure 6: Inactivation of the cuneate nucleus abolished responses to chin stimulation in the deafferented parts of area 3b in monkey LM59. ( a ) Outline drawings of the cuneate nucleus from three different rostrocaudal coronal sections of the medulla showing locations of the receptive fields in 10 different electrode penetrations. Note extensive responses to stimulation on the chin. ( b ) Approximate locations of the electrode tips in area 3b (see ‘Methods’). For reference somatotopic map derived separately is placed in the background, which also shows expansion of the chin responsive region in the deafferented hand cortex. ( c ) A reconstruction of the spinal cord in a coronal plane showing the extent of the dorsal column lesion. ( d ) PSTH and waveforms of neuronal responses to stimulation of the chin at a recording site marked by deep red dot in the cuneate nucleus (blue) before lidocaine infusion. Two responsive units are clearly discernable. ( e ) PSTH showing multiunit responses in area 3b to chin stimulation at recording sites shown in ‘ b ’ before infusion of lidocaine in the cuneate nucleus. ( f ) Location of the stimulation site on the chin (black dot) during recordings for graphs shown in panels ‘ d ’, ‘ e ’, ‘ g ’ and ‘ h ’. ( g ) PSTH showing that neuronal responses in the spinal trigeminal nucleus were not affected by injection of lidocaine in the adjacent cuneate nucleus. ( h ) Neuronal responses at the same sites as for recordings shown in ‘ e ’ after lidocaine infusion. Responses in the normal chin region were intact, while those in the deafferented hand cortex were abolished. The x -axis range is from 100 ms before the stimulation onset (arrow) to 100 ms post-stimulus onset for ‘ e ’ and ‘ h ’, and from 400 ms pre-stimulus onset to 400 ms post-stimulus onset for ‘ d ’ and ‘ g ’. Scale bars, 1 mm. For other conventions see Figs 2 , 4 and 5 . Full size image We then placed an array of electrodes in area 3b. The lateral-most electrode of the array was in the normal chin region and the medial three electrodes were in the deafferented hand cortex, one of which was near the hand-face border. Another microelectrode was placed in the cuneate nucleus and the chin was stimulated at 1 Hz as described above. After recording neuronal responses simultaneously from area 3b and the cuneate nucleus ( Fig. 6d,e and f ), we inactivated neurons in the cuneate nucleus by injection of lidocaine. Lidocaine was injected at four rostrocaudal sites at a depth of 800 μm from the surface of the medulla. At each of the two caudal sites 4 μl of lidocaine, and at the two rostral sites 3 μl of lidocaine, was injected. Post-inactivation recordings were started 17 min after the last injection. We verified that neurons in the adjacent trigeminal nucleus continued to respond to stimulation of the chin during the period when the cuneate nucleus was inactivated ( Fig. 6g ). Recordings from the electrodes in the cortex showed that neurons in the normal chin representation continued to respond to stimulation of the chin as before; whereas neurons recorded from the electrodes in the expanded chin representation no longer responded to the chin stimulation ( Fig. 6h ). These data clearly show that large-scale expansion of the chin inputs into the deafferented hand region of area 3b depends on inputs from the reorganized cuneate nucleus of the brainstem. Brain reorganization following deafferentations due to injuries has been most extensively studied in the cortex because neocortex is regarded as the most plastic part of the mammalian brain and it is easily accessible to experimental investigations. However, our results presented here unequivocally show that expansion of chin inputs into the deafferented hand region of area 3b is due to changes taking place in the brainstem nuclei. If the information flow from the reorganized cuneate nucleus of the brainstem is interrupted, the reorganized cortex becomes silent. The possibility that sprouting from the spinal trigeminal nucleus into the cuneate nucleus likely mediates face expansion was first suggested by Pons and others [5] . It has been a favourite hypothesis to explain large-scale brain reorganization for many reasons. One, the brain reorganization is seen as early as 6–10 months post-injury [1] , [22] , [32] . Since topographic representations in the small brainstem nuclei are highly compressed, growth for only a short distance would be adequate for the large-scale reorganization (~0.2–2 mm in the medulla versus 7–14 mm in area 3b). Two, reorganization results in expression of chin inputs in the deafferented hand region [2] , [3] ; since chin inputs in the spinal trigeminal nucleus lie adjacent to the cuneate nucleus [22] , [33] , [34] , they are most likely to sprout into the deafferented cuneate nucleus [5] , [13] , [35] . Moreover, growth of chin inputs from the trigeminal nucleus into the cuneate nucleus has been reported in monkeys with dorsal column injuries [22] . Finally, because of high fidelity of connections between isorepresentations along the somatosensory pathway, expansion of chin inputs into the cuneate nucleus will automatically reflect as chin expansion in the deafferented hand regions of the somatosensory thalamus and cortex [13] ( Fig. 1 ). Our data also rule out thalamic-mediated plasticity, because, if reorganization in the VPL nucleus was due to expansion of the chin inputs from ventroposterior medial nucleus, inactivation of the cuneate nucleus would not completely eliminate the emergent chin expansion in the cortex. Possibility of other novel connections that could reactivate the hand region of area 3b viz. growth of collateral projections from the trigeminal nucleus to VPL or from VPM to the hand cortex ( Fig. 1d ) is also similarly ruled out. More restricted deafferentations such as nerve injuries, amputations or transection of some of the dorsal roots from the hand result in more limited cortical plasticity in adult primates. In such cases, the reorganization is restricted to the representation of the same body part. The reorganization is also observed in the cuneate nucleus and VPL of the thalamus [30] , [36] , [37] , [38] . The nature of reorganization is broadly similar across these sites, although the fine details vary as discussed below. Thus, it remains likely that plasticity following injuries in the somatosensory system is due to changes in the brainstem nuclei, which are propagated upstream. There are reports of sprouting in the spinal cord as well as the cuneate nucleus following therapeutic amputations of the arm [39] and restricted transection of the dorsal roots from the hand [40] . However, it is not known whether the cuneate nucleus reorganization is critical for expression of the thalamic and cortical plasticity in these cases. Similarly, no causal relationship between cortical growth and plasticity was shown in monkeys with forelimb amputations [25] . Although change in one part of the brain has wide-ranging effects throughout the system, details of reorganization at each level in the pathway could be different due to influence of local mechanisms. Differences in the nature of reorganization between area 3b and the cuneate nucleus after median and ulnar nerve injuries [30] , VPL and area 3b after chronic spinal cord injuries [2] or after limb amputations [37] have been described. These could be due to specific nature of the ascending projections, local intrinsic circuitry and the feedback network at each level. For example, in the primary visual cortex matched binocular lesions of retina result in filling-in of the resulting scotoma by the surrounding visual field, a change of 6–8 mm, which is mediated by sprouting of horizontal cortical connections [23] , [24] . After such injuries, unlike the somatosensory system, no reorganization was observed subcortically in the lateral geniculate nucleus [41] . Furthermore, deafferentation-induced mechanisms operating at different levels can further modify details of the reorganization. The mechanisms can include unmasking and growth of pre-existing connections, changes in neurotransmitter levels and withdrawal of terminals due to deafferentation [20] , [27] , [36] , [42] , [43] , [44] . Brain reorganization has been proposed to cause phantom sensations [7] , [8] , [9] and mediate therapy-induced recoveries by potentiation of uninjured pathways [10] . Our results from these experiments establish critical role of expansion of chin inputs in the cuneate nucleus for expression of cortical plasticity and suggest possible therapeutic target sites to clinically control brain reorganization. Animals Five adult male macaque monkeys were used in these experiments. Three of the monkeys, LM59, LM76 and LM105, were Macaca mulatta, and two, LM49 and LM95, were Macaca radiata . Monkey LM105 was used previously for other experiments [45] . Monkeys LM49 and LM95 were 13.5 and 12.7 years old at the time of the spinal cord lesion. Monkeys LM59, LM76 and LM105 were adults and weighed 11.3 kg, 9.3 kg and 7.3 kg at the time of the lesion. Exact age of these monkeys is not known since they were not born in the animal facility. The animal protocols were approved by the Animal Ethics Committee of the National Brain Research Centre, and the Committee for the Purpose of Control and Supervision of Experiments on Animals (CPCSEA), Government of India. The procedures conformed to NIH guidelines. Dorsal column lesions The animals were anaesthetized using a mixture of ketamine (8 mg kg −1 , IM) and xylazine (0.4 mg kg −1 , IM). Further supplemental doses of the anaesthetics were given at one-tenth of the initial dose during the course of surgery as required. Procedures for making lesions of the dorsal columns have been described in detail before [2] , [3] . In brief, the dorsal neck and the upper back were prepared for surgery, and a midline incision was made in the skin. The muscles were retracted to expose the vertebrae. A small laminectomy was done, dura was incised and the dorsal columns were sectioned unilaterally from midline to the point of entry of the dorsal roots using a pair of sharp fine forceps, taking care to minimize damage to the surface blood vessels. The dura was folded back in place, and the spinal cord was covered with gel foam. Muscles and skin were sutured in layers, and the animals were allowed to recover from anaesthesia and monitored carefully. The animals were given antibiotics, analgesics and dexamethasone for 5 days post surgery [2] . Heart rate, blood oxygenation levels and core body temperature were continuously monitored during the entire procedure. During the recovery period, the animals were carefully monitored for food and fluid intake. No complications were observed, and the recoveries were uneventful. Multiunit mapping Topography of the primary somatosensory cortex, area 3b, was determined using standard multiunit electrophysiological techniques [3] . Receptive fields of neurons were determined at 300–400 μm intervals as the electrode was advanced down the posterior bank of the central sulcus. At each recording site, the entire body was thoroughly explored for neuronal responses to light tactile stimulation, taps and movements of joints and muscles. The electrode penetrations were spaced to cover the entire hand and face regions of area 3b. In monkey LM76, 219 recording sites were mapped in 18 penetrations, and in monkeys LM95 and LM105 receptive fields for neurons at 249 and 220 sites were determined in 18 and 17 penetrations, respectively. Finally, in monkeys LM49 and LM59, 21 and 22 penetrations were made and receptive fields determined at 289 and 240 recording sites, respectively. For mapping the brainstem nuclei in monkeys LM49 and LM59, the head of the animal was stabilized in a stereotaxic frame with the neck in a dorsiflexed position. A midline incision was made over the medulla, and the neck muscles were retracted. A small part of the occipital bone overlying the cerebellum was removed carefully using a pair of rongeurs. Ventral most part of the vermis was removed by subpial aspiration for better access to the medulla. Dura over the fourth ventricle was reflected to expose the brainstem up to 1.2 mm rostral to obex. For mapping, the microelectrode was positioned approximately perpendicular to the dorsal surface of the medulla. The electrode was advanced using hydraulic microdrive (David Kopf Instruments, CA, USA), and receptive fields of neurons were determined every 100 or 200 μm along the dorsoventral axis. In monkey LM49 we mapped receptive fields at 55 recording sites in 11 electrode penetrations, while in monkey LM59 we mapped 110 sites in 22 electrode penetrations. The penetrations were made with a goal to cover the entire cuneate nucleus, large parts of the spinal trigeminal nucleus and parts of the gracile nucleus. To identify the orientations and locations of the electrode tracks in area 3b and the brainstem nuclei, few tracks were marked by passing a current of 10 μA as the electrode was slowly withdrawn. In some of the monkeys, we also marked few tracks by coating the electrode with fluorescent dye, DiI before insertion ( Fig. 7 ; see [2] ). 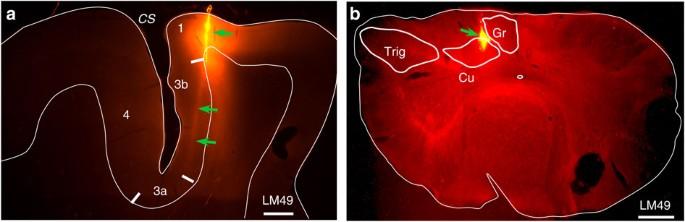Figure 7: Examples of electrolytic lesions and fluorescently labelled electrode tracks. (a) A photomicrograph through the central sulcus (CS) showing an electrode track (green arrows) marked by coating the electrode with DiI before insertion in area 3b of monkey LM49. The top part of the track is highly fluorescent, while the bottom part is faint because it was mainly located in the adjacent section. Borders of areas 1, 3b, 3a and motor area 4 were drawn with the help of adjacent Nissl and cytochrome oxidase (CO)-stained sections. (b) A composite of photomicrographs through the medulla of monkey LM49 showing fluorescent track (green arrow) made in a manner similar to ‘a’. Outlines of the spinal trigeminal nucleus (Trig), cuneate nucleus (Cu) and the gracile nucleus (Gr) are shown. Scale bars, 1 mm. Figure 7: Examples of electrolytic lesions and fluorescently labelled electrode tracks. ( a ) A photomicrograph through the central sulcus (CS) showing an electrode track (green arrows) marked by coating the electrode with DiI before insertion in area 3b of monkey LM49. The top part of the track is highly fluorescent, while the bottom part is faint because it was mainly located in the adjacent section. Borders of areas 1, 3b, 3a and motor area 4 were drawn with the help of adjacent Nissl and cytochrome oxidase (CO)-stained sections. ( b ) A composite of photomicrographs through the medulla of monkey LM49 showing fluorescent track (green arrow) made in a manner similar to ‘ a ’. Outlines of the spinal trigeminal nucleus (Trig), cuneate nucleus (Cu) and the gracile nucleus (Gr) are shown. Scale bars, 1 mm. Full size image Cortical inactivation Normal chin region in area 3b was inactivated in monkeys LM76, LM95 and LM105. Lidocaine (4%, Neon Laboratories Ltd, India) was infused approximately 0.8–1.5 mm from the hand-face border using a fine capillary tube [46] , [47] . The capillary tube was attached to a 1-ml syringe loaded with lidocaine and fitted to a syringe pump (Harvard Apparatus, MA, USA). The glass capillary was held in place by a custom-built device that could also hold up to two independently moveable electrodes. This device facilitated simultaneous lidocaine infusion and recording of neuronal activity in the vicinity of the capillary to monitor the extent of inactivation. The infusion protocol consisted of an initial bolus of 10–15 μl at a rate of 4 μl min −1 , followed by continuous infusion at a slower rate (0.5 μl min −1 ), which was maintained throughout the mapping and recording sessions. A second bolus was given 30–40 min later. The rate of infusion and the location of the injections were standardized from our experiments in a normal monkey to ensure complete inactivation of the normal chin region without affecting the cortex medial to the hand-face border. The recordings were started when no chin responses could be evoked in the normal chin region. Cuneate inactivation The cuneate nucleus was inactivated in monkeys LM49 and LM59 using a capillary tube as described above. Lidocaine (4%) was injected at four sites spanning 3 mm rostrocaudally at a depth of 700–1,500 μm from the medullary surface. At each site 2 or 4 μl lidocaine was injected at the rate of 4 μl min −1 . Care was taken while selecting the site and volume of injections [46] to avoid spread of lidocaine to the adjacent spinal trigeminal nucleus and the ventrally located respiratory centres. Evoked neuronal responses to tactile stimulation of the chin were recorded simultaneously from the normal chin and deafferented hand regions of area 3b and the brainstem nuclei. Quantification of neuronal responses Punctate stimuli were delivered on the chin or the hand by a Chubbuck type electromechanical stimulator (CS-525 Tactile Stimulator, Cantek Metatron Associates, USA). The train of stimuli consisted of periodic skin contact with a probe (tip diameter, 5 mm) for 10 ms every 1 s or for 25 ms every 2 s. For stimulation of the chin, hairs were trimmed to about 1 mm length to avoid unwanted spread of the stimulus. In a single recording session, 300 stimuli were delivered. Recordings were made using both a single electrode and custom-built multi-electrode arrays of parylene-coated tungsten microelectrodes (1 MΩ at 1 kHz, Microprobe, MD, USA). The extracellular voltage signals were acquired using Multichannel Acquisition Processor (MAP; Plexon, Dallas, Texas, USA). The signals were band-pass filtered between 150 Hz and 8 kHz, digitized at 40 kHz and stored for offline sorting and analyses. The spike data were sorted into multiunit clusters using Plexon Offline Sorter (Plexon, Dallas, Texas, USA). Timestamps of the spikes and the stimulus events were used to plot peristimulus time histograms using Neuroexplorer software (version 4.095; Plexon, Dallas, Texas, USA). The data were exported to MATLAB (The Mathworks, Natick, MA, USA) for further analyses. The spike timings were binned into 1-ms bins to plot the histograms. The histograms were smoothed with a boxcar filter (filter width, three bins). Background activity was defined as the mean firing rate during the 100 ms period before onset of the stimulus. Neurons were considered to be responsive (that is, a peak was present) when value of three consecutive bins exceeded the background activity plus 3 s.d. Peak firing rate was the highest bin value during the response period. Statistical analysis Mann–Whitney rank sum test was used to statistically compare peak firing rates of neurons in response to chin stimulation in the expanded chin representation of monkeys LM76, LM95 and LM105 before and after inactivation of the normal chin representation in area 3b. In monkeys LM49 and LM59, peak firing rates of neurons in the normal chin representation of area 3b were statistically compared using Mann–Whitney rank sum test before and after inactivation of the cuneate nucleus with lidocaine. The differences were considered to be statistically significant if P <0.05. Histology After completion of the entire experiment, the monkeys were perfused transcardially as described before [3] , [32] . After perfusion, the brain was removed, the cortex separated from the subcortical tissue, blocked and cryoprotected in 30% sucrose. Cortex surrounding the central sulcus was blocked, frozen and cut into 50-μm thick sections on a sliding microtome in a plane perpendicular to the central sulcus, which is slightly off the parasagittal plane. Series of adjacent sections from the cortex were stained for Nissl substance, cytochrome oxidase (CO) activity [48] and acetylcholine esterase activity [49] to help identify electrode tracks and to determine architectonic boundaries between different cortical areas. One series of sections was mounted unstained to locate fluorescently labelled electrode tracks ( Fig. 7a ). For monkey LM59, the cortex was flattened and cut parallel to the pial surface, and alternate sections were stained for myelin [2] . Medulla was cut coronally into 36- or 40-μm-thick sections. A series of alternate brainstem sections was stained for cytochrome oxidase activity to visualize boundaries of nuclei and the electrolytic lesions. The second series was mounted unstained to examine fluorescently labelled electrode tracks ( Fig. 7b ). The spinal cord was also removed, cryoprotected as above and cut at 40- or 50-μm-thick sections in a horizontal plane. The sections were mounted unstained and observed under dark-field illumination for reconstruction of the lesion site (see below). Reconstruction of the somatosensory map in area 3b Neuronal responses were qualitatively classified based on the kind of the stimulus required into those requiring light touch, hair stimulation, taps or hard taps, each of which was represented by a different symbol ( Fig. 2 ). The somatotopic map was reconstructed [32] using Canvas X software. The map was overlaid on a 3-dimensionsal (3D) reconstruction of the posterior bank of the central sulcus made from the histological sections. The 3D reconstruction was done from drawings of the sections digitized by scanning and using serial section manager of Neurolucida software (Microbrightfield, VT, USA). The somatotopic map was aligned to this 3D view with the help of the electrolytic lesions and the fluorescent tracks. Reconstruction of somatotopic map in the cuneate nucleus The progression of receptive fields along the dorsoventral axis for each electrode penetration was first reconstructed as described for area 3b. These reconstructions were transferred to outline drawings of the sections of the medulla from appropriate rostrocaudal level. The alignment was done with the help of electrolytic lesions and fluorescent tracks as described above. Reconstruction of the spinal cord lesion Drawings of the spinal cord sections in the region of the lesion were made using a microscope equipped with camera lucida. The maximal extent of the lesion and boundaries of the white matter and grey matter were measured and plotted on a graph paper for each section. The corresponding boundaries were joined to visualize the extent of the lesion in a coronal view of the spinal cord [50] . How to cite this article: Kambi, N. et al. Large-scale reorganization of the somatosensory cortex following spinal cord injuries is due to brainstem plasticity. Nat. Commun. 5:3602 doi: 10.1038/ncomms4602 (2014).